The impact of asymmetrical light input on cerebral hemispheric specialization and interhemispheric cooperation Hemispheric specialization potentially provides evolutionary advantages by enhancing cognitive capacities. However, separation of function might be advantageous only with the presence of commissural systems allowing for efficient information exchange and cooperation between the hemispheres. Here we investigate hemispheric cooperation in pigeons as they possess an asymmetrically organized visual system that develops in response to biased ontogenetic light stimulation. This allows comparison of the integration capacities of lateralized (light-incubated) and non-lateralized (dark-incubated) animals. We show that pigeons integrate information learnt separately with each hemisphere when confronted with a transitive reasoning task that they cannot solve with the knowledge of one hemisphere alone. Impairments in dark-incubated birds demonstrate that this ability depends on asymmetrical embryonic light stimulation. Our study provides for the first time direct evidence that lateralized environmental experience not only induces hemispheric specialization, but also affects the efficiency of interhemispheric crosstalk. Environmental factors can influence the tight interplay between the hemispheres, which in turn determines cognitive abilities. Cerebral lateralization refers to the differential functional organization of the left and right hemispheres, which therefore have different roles in the mediation of behaviour and emotional or cognitive processing [1] . However, although cerebral hemispheres may independently process information in their own specialized ways, interhemispheric communication systems have to merge this information to acquire a complete representation of the environment, or to combine hemispheric-specific knowledge for optimal cognition. Accordingly, even profoundly lateralized cognitive functions, such as speech processing, benefit from efficient interhemispheric communication [2] . On the other hand, developmental disorders like autism [3] , dyslexia [4] or schizophrenia [5] are characterized by untypical cerebral lateralization patterns as well as structural peculiarities of the corpus callosum that are related to cognitive impairments [6] , [7] , [8] , [9] , [10] . Although several studies suggest a relationship between functional lateralization and structural organization of commissural systems, for example [11] , [12] , the functional and developmental relationships remain controversial [13] . One may suppose enhanced integration of information that was processed by specialized hemispheres, at least in tasks requiring the expertize of both hemispheres. However, such a relation is not yet substantiated, because direct proof is difficult to obtain in humans or other mammals, owing to the quick information exchange via the corpus callosum. Moreover, an experimental analysis requires models allowing for experimental manipulations of the degree of cerebral asymmetries. The avian visual system is such a model. Vision is highly developed in many birds and subserves complex cognitive abilities [14] , [15] . Comparable to humans, the two brain halves of chicks or pigeons contribute differently to cognitive challenges and display several structural and functional left–right differences [16] , [17] , even though birds do not possess a corpus callosum-like forebrain commissure. These hemispheric specializations can be easily tested just by occluding one eye with an eye cap as the avian optic nerves cross completely. However, pigeons exhibit a quantitative advantage of using both eyes as compared with monocular performances [18] and this advantage increases with task complexity [19] . Accordingly, hemispheric-specific information is exchanged and integrated to acquire optimal visuomotor responses. This functional organization shows that the presence of a corpus callosum-like forebrain commissure is not a prerequisite neither for the generation of hemispheric asymmetries nor for the ability to integrate information, as discussed in human research [13] , [20] . Binocular performance, in turn, correlates with the degree of visual lateralization [18] and strongly lateralized chicken demonstrate a better ability to carry out representational learning than less-lateralized individuals [21] . Visual asymmetries develop in response to asymmetrical light stimulation as indicated by the absence of asymmetrical differentiation processes in dark-incubated birds [16] , [22] , [23] . This allows us to compare the capacity of hemispheric cooperation in lateralized and non-lateralized birds, in order to investigate the impact of ontogenetic experience on the interrelations between hemispheric specialization and integration. To this end, we confronted normal (lateralized) and dark-incubated (non-lateralized) pigeons with a cognitive problem that cannot be solved with the knowledge of one hemisphere alone, but that requires interhemispheric cooperation. Similar to several animal species [17] , [21] , pigeons are able to detect a relation between two items that are never presented together before. Thus, they can rank pattern after learning to discriminate overlapping pairs of stimuli according to transitive inference logic [24] . In this report, we adopted a transitive reasoning paradigm by providing each eye/hemisphere of a pigeon with only half of the information required to establish a transitive line. We demonstrate that normal, but not dark-incubated pigeons, successfully pass the critical integration task, suggesting that lateralized visual experience not only induces hemispheric specialization but also affects the efficiency of interhemispheric cooperation. Monocular and binocular colour discrimination We adopted a transitive inference task by training pigeons to discriminate four pairs of stimuli A+B−, B+C−, C+D− and D+E− presented as differentially coloured grit [24] . As monocular training enables to restrict information primarily to the contralateral hemisphere, we parcelled the stimulus pairs out ( Fig. 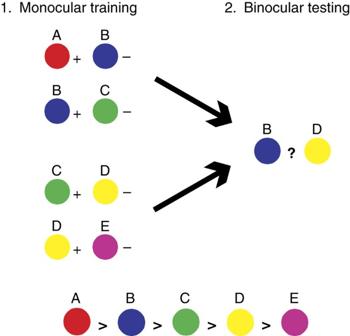Figure 1: Rational of the transitive inference task. Pigeons were trained to discriminate four overlapping pairs of colour stimuli A+B−, B+C−, C+D−and D+E− representing a linear hierarchy. Thereby each eye learnt to discriminate only two of the pairs. To analyse transitive responding, subsequent binocular test sessions were conducted confronting the animals with novel, non-rewarded stimulus pairs, with BD as the most relevant one. 1 , Table 1 ). Each eye learned to discriminate only two premise colour pairs so that inferences about hierarchical ranking order of the learnt stimuli (A>B>C>D>E) required integration of knowledge from both hemispheres. This ability was tested after monocular training when the animals were confronted with new colour combinations while seeing with both eyes. Figure 1: Rational of the transitive inference task. Pigeons were trained to discriminate four overlapping pairs of colour stimuli A+B−, B+C−, C+D−and D+E− representing a linear hierarchy. Thereby each eye learnt to discriminate only two of the pairs. To analyse transitive responding, subsequent binocular test sessions were conducted confronting the animals with novel, non-rewarded stimulus pairs, with BD as the most relevant one. Full size image Table 1 Detailed training procedure. Full size table After training, normal as well as dark-incubated animals achieved comparable choice accuracies for all colour pairs without any difference between the pairs or between the left- and right-eye seeing conditions ( Fig. 2 ). This indicates that the two groups displayed comparable associative learning abilities [24] with both hemispheres. 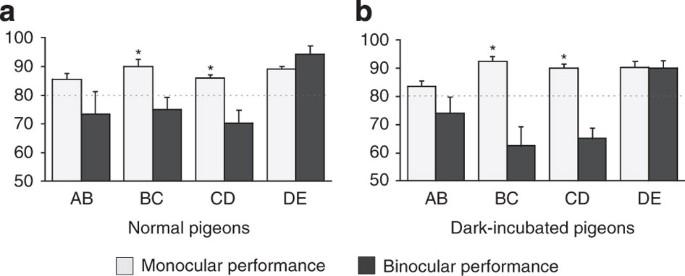Figure 2: Performance in discriminating trained colour pairs. Monocular (training) and binocular (testing) choice accuracies of trained colour pairs in normal (a) and dark-incubated pigeons (b). In both groups, binocular discrimination of DE differed significantly from the other pairs and binocular discrimination accuracies were significantly reduced compared with monocular ones for pairs BC and CD. Bars represent ±s.e.m. of the data points; dashed line indicates the 80% learning criterion (*P<0.05 according to Wilcoxon tests). Figure 2: Performance in discriminating trained colour pairs. Monocular (training) and binocular (testing) choice accuracies of trained colour pairs in normal ( a ) and dark-incubated pigeons ( b ). In both groups, binocular discrimination of DE differed significantly from the other pairs and binocular discrimination accuracies were significantly reduced compared with monocular ones for pairs BC and CD. Bars represent ±s.e.m. of the data points; dashed line indicates the 80% learning criterion (* P <0.05 according to Wilcoxon tests). Full size image Choices during critical binocular testing were analysed by non-parametric Friedmans analysis of variances (ANOVAs). In contrast to monocular training performances, choice accuracies differed between learnt colour pairs (normal birds: χ 2 ( n =14, df=3)=13.081, P =0.005; dark-incubated: χ 2 ( n =8, df=3)=4.671, P =0.021). In both groups, binocular discrimination performances decreased for all colour pairs except for DE, which was significantly better discriminated than the other pairs (Wilcoxon: P <0.05 for all comparisons, Fig. 2 ). Thus, interestingly, an end-anchor effect emerged when seeing with both eyes despite equal monocular learning performances. Moreover, binocular discrimination of colour pairs BC and CD was significantly reduced compared with monocular performances (Wilcoxon: P <0.05, Fig. 2 ). In dark-incubated birds, discrimination of pair BC did not even clearly differ from chance anymore (Wilcoxon: P =0.07). However, there was no difference in discrimination accuracy for any of the training pairs between the two groups. Pairs BC and CD included colour C, the colour with complementary reward value for the two eyes. This suggests that the transfer of monocular knowledge on binocular situations is problematic, when monocular experiences represent conflicting information. However, these problems might affect integration of hemispheric-specific information differently in normal and dark-incubated pigeons as indicated by differences in choice behaviour when confronted with the unlearnt test pairs. Binocular transitive inference performance During critical testing, normal animals decided more often for the transitively correct colour, although confidence levels differed between the colour pairs (Friedmans ANOVA: χ 2 ( n =14, df=5)=15.833, P =0.007; Fig. 3a ). Comparison between correct and false decisions yielded a well-above-chance transitive responding for all extinction trials, even for colour B, in the most critical test pair BD (Wilcoxon: P <0.01 for all colour pairs). This choice behaviour demonstrated that the animals ranked the colour stimuli according to the transitive line, which required combination of knowledge from both hemispheres. In this regard, it was insignificant which hemisphere learnt the beginning or end pairs of the transitive line ( Fig. 3b ). 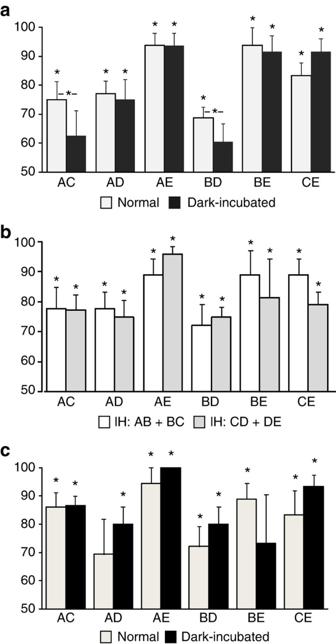Figure 3: Binocular transitive responding of normal and dark-incubated pigeons. Mean choice percentages for the transitively correct colours within the six test pairs during binocular test sessions of normal (n=14) and dark-incubated (n=8) pigeons after monocular learning indicated correct transitive responding only for normal animals (a). Note that, accordingly, the performance of AC and BD differed significantly between groups. Transitive responding in normal pigeons did not depend on hemispheric-specific allocation of training pairs as shown by the comparison of binocular transitive performance of animals, which learnt beginning (AB, BC;n=6) or end pairs (CD, DE,n=8) of the transitive line with the right eye/left hemisphere (lH), respectively (b). (c) After binocular training, normal (n=6) as well as dark-incubated (n=6) animals displayed a significant above chance transitive responding for nearly all colour pairs with exception of pair AD in normal pigeons (Z=1.826,P=0.067) and BE in dark-incubated birds (Z=1.753,P=0.0796). This was owing to one animal in each case that discriminated only these colour pairs particularly low. These data confirmed the results of Siemannet al.24for normal pigeons and demonstrated that dark-incubated pigeons could rank colour items according to transitive inference logic after binocular training. Bars represent ±s.e.m. of the data points (*P<0.05 according to Wilcoxon, or Mann–Whitney U-test, respectively). Figure 3: Binocular transitive responding of normal and dark-incubated pigeons. Mean choice percentages for the transitively correct colours within the six test pairs during binocular test sessions of normal ( n =14) and dark-incubated ( n =8) pigeons after monocular learning indicated correct transitive responding only for normal animals ( a ). Note that, accordingly, the performance of AC and BD differed significantly between groups. Transitive responding in normal pigeons did not depend on hemispheric-specific allocation of training pairs as shown by the comparison of binocular transitive performance of animals, which learnt beginning (AB, BC; n =6) or end pairs (CD, DE, n =8) of the transitive line with the right eye/left hemisphere (lH), respectively ( b ). ( c ) After binocular training, normal ( n =6) as well as dark-incubated ( n =6) animals displayed a significant above chance transitive responding for nearly all colour pairs with exception of pair AD in normal pigeons ( Z =1.826, P =0.067) and BE in dark-incubated birds ( Z =1.753, P =0.0796). This was owing to one animal in each case that discriminated only these colour pairs particularly low. These data confirmed the results of Siemann et al . [24] for normal pigeons and demonstrated that dark-incubated pigeons could rank colour items according to transitive inference logic after binocular training. Bars represent ±s.e.m. of the data points (* P <0.05 according to Wilcoxon, or Mann–Whitney U-test, respectively). Full size image In dark-incubated pigeons, choices also differed between colour pairs (Friedmans ANOVA: χ 2 ( n =8, df=5)=26.901, P =0.00001; Fig. 3a ). Comparison between correct and false decisions demonstrated significantly correct responses in pairs, which included consistently rewarded (A) or non-rewarded (E) colours ( Fig. 3a ). In contrast, the animals did not show a significant difference between correct and false responses for pair AC (Wilcoxon: Z =1.258, P =0.208). This pair combined the two colours with highest reward value for each eye and therefore, might provide conflicting information if the colours were not ranked along the transitive line. As the animals also failed to respond correctly to pair BD (Wilcoxon: Z =1.214, P =0.225), these results clearly demonstrate that the birds did not respond based on relational learning. Moreover, choice behaviour for these two colour pairs differed substantially from that of normal animals (Mann–Whitney U-tests: AC: Z =1.929, P =0.055; BD: Z =2.023, P <0.05; Fig. 3a ). Failure to integrate information of the hemispheres is presumably what caused this impairment, as dark-incubated pigeons displayed transitively correct choices after binocular training ( Fig. 3c ). Our data clearly show that normal pigeons are able to integrate information from the two hemispheres to solve a higher cognitive task. We cannot definitely decide if choices during critical testing are based on relational or associative information [25] , [26] , but both mechanisms require comparison and integration of hemispheric-specific knowledge to make inference judgements. However, cognitive demands differ between test pairs and may therefore involve different modes of interhemispheric cooperation. The easiest pair AE can be discriminated purely based on associative memory although each hemisphere has direct experience only with one of the colours. Correct choices require comparison of reward values (A always, E never rewarded), and here normal and dark-incubated animals did not differ in performance. A more complex cognitive process underlies correct decisions for colour pairs including ambiguous information about reward values within, or between, the hemispheres. These are pairs AC and BD, and only these pairs revealed differences in choice behaviour between the groups. Pair AC combined colours representing highest value for the two eyes and colour stimuli in BD were equally often rewarded as well as non-rewarded. Choice behaviour in normal animals makes it likely that transitively correct decisions rely on mechanisms that detect an ordered hierarchy after combination of hemispheric-specific knowledge [24] , [27] . This ability goes beyond the integration of mnemonic material in commissurectomized monkeys [28] or voluntary attention, in split-brain patients [29] , although pigeons lack a corpus callosum-like forebrain commissure, too. This cognitive ability was profoundly impaired in dark-incubated pigeons. Thus, efficiency of interhemispheric crosstalk depends on asymmetrical light input during embryonic development. Asymmetrical experience does not only induce hemispheric specialization, but also controls how the hemispheres interact to integrate information for higher cognition. The structural basis for this kind of hemispheric cooperation is still speculative. On the one hand, ascending visual fibres cross within the diencephalic supraoptic decussation, and interocular transfer of pattern, brightness or colour discrimination depends on the integrity of this commissure [30] , [31] , [32] . Accordingly, information exchange that is critical for correct choices might be mediated during primary visual processing. On the other hand, mainly inhibitory subcortical or brainstem commissures regulate hemispheric dominance, cooperation and switching [16] , [33] as shown in the avian song system [34] or for lateralized visuomotor processing in pigeons [16] , [33] , [35] . Although these systems do not directly mediate information transfer, they may control the degree of information exchange and, in consequence, interhemispheric integration. In pigeons as in other birds, asymmetrical light stimulation before and after hatching biases differentiation of the ascending visual pathways. Despite the complete crossing of the optic nerves [36] , unilateral modulation of visual input affects neuronal circuits on both brain sides [37] , [38] . Such bihemispheric effects require the action of commissural systems, which mediate the balance of left- and right-hemispheric developmental processes and which presumably stabilize induced left–right differences [16] , [37] . It is conceivable that these developmental interactions also affect the efficiency of the interhemispheric crosstalk itself [39] , which in turn limits cognitive abilities that need the integration of information from both hemispheres. Reduced cerebral lateralization alone does not necessarily lead to minor cognition [21] as normal and dark-incubated pigeons display comparable transitive reasoning after binocular training. Deficits may only emerge when information of one hemisphere is not sufficient to solve a cognitive problem. These results suggest that cognitive impairments as observed in developmental or psychiatric disorders might also be only fully comprehensible by an understanding of abnormal interhemispheric communication systems, although genetic and/or environmental factors may primarily cause aberrations of intrahemispheric circuits [6] , [7] . Animals Fourteen normal adult domestic pigeons ( Columba livia ) from local breeders as well as eight adult dark-incubated animals from lab-own breeding pairs [23] served as subjects for an operant transitive inference experiment. The animals were housed in individual cages and were kept food-deprived to ∼ 80% of their free-feeding weight throughout the experiment. The study was carried out in compliance with the European Communities Council Directive of November 24, 1986 (86/609/EEC) and the specifications of the German law for the prevention of cruelty to animals. Rational of the task The transitive inference task was designed as simultaneous colour discriminations whereby pigeons were trained to discriminate four overlapping pairs of stimuli A+B−, B+C−, C+D− and D+E− that represent a linear hierarchy in which responses to higher-ranked stimuli were rewarded ( Fig. 1 ). Letters stood for five varieties of non-toxic aquarium grit differing in particle colour and size (green, blue, brown, pink and yellow). A grain of maize buried under the positive grit rewarded correct choices [24] . Each eye learnt to discriminate two colour pairs whereby we minded that stimulus ordering and presentation did not correlate with any physical gradient or cognitive processing asymmetries. Accordingly, several parameters were controlled. First, we controlled for the order of the transitive line. The coloured grits were presented in the pairs AB, BC, CD and DE. To control for any spontaneous grit preferences, the correspondence of the various grits to the letters was reversed for half of the birds. Second, we controlled for hemispheric-specific learning. As evidences from chicken experiments suggest different transitive reasoning abilities of the left and right hemisphere [17] , it might have been critical which of the eyes learnt the beginning or end pairs of the transitive line. Therefore, attribution of the colour pairs was balanced between the eyes. Third, we controlled for biased frequency design. To avoid the emergence of an end-anchor effect that might allow explaining choices with simple associative learning, the presentation frequencies of the training pairs were biased according to Siemann et al . [24] To this end, training was started with the more difficult middle pairs BC and CD as these pairs contain colours that were rewarded as well as non-rewarded. These pairs were also trained with higher frequency than the two easier pairs AB and DE. As choice accuracies obtained at the end of training were equal for all pairs (all above 80%), the design was successful in avoiding an end-anchor effect. Colour discrimination training Daily sessions consisted of 30 trials while seeing with the left or right eye only. The coloured grits were presented in two plastic cups (4 cm in diameter and 6 cm deep) set side-by-side into a plastic trough that was placed below the central opening of the home cages. The trial-to-trial left–right position of the colour stimuli varied quasi-randomly. A correct choice was recorded when the pigeon pecked into the positive (baited) grit and the animal then was allowed to find the hidden grain. Searching among the non-baited grit was classified as an error choice and the trial ended by removing the box. Only during the early training phase, a pigeon could switch to the positive grit to find the reward grain. Training began with the more difficult colour pairs BC and CD [24] (for details see Table 1 ). After reaching the learning criterion of 80% correct choices in three consecutive sessions for an individual eye, the second pairs (AB or DE, respectively) were introduced. Colour pairs were presented in runs, first consisting of ×20 (BC or CD) + ×10 (AB or DE), then of ×2 (×10 BC/CD + ×5 AB/DE) repeated trials. During the last training sessions, 20% of the training trials remained unrewarded to exclude that the pigeons' discriminative behaviour based upon unintended cues such as grain visibility or smell and to prepare the animals for the extinction trials. Transitive inference test Subsequently, six test sessions were conducted under binocular seeing conditions with novel, non-rewarded stimulus pairs AC, AD, AE, BD, BE and CE randomly interspersed among the rewarded training pairs. Choices were recorded when the pigeon pecked into the grit closest to the beak. We analysed if animals performed according to transitive inference logic. To this respect, the most critical test pair was BD because the component stimuli served equally often as rewarded and as non-rewarded stimuli in the premise training pairs. Thus, their value could only be estimated in relation to the other colours, and hence after ranking along the transitive line. This required integration of information as each eye/hemisphere had direct experience with only half of the colours. Accordingly, correct decision for B indicated successful transitive inference conveyed by hemispheric cooperation. How to cite this article: Manns, M. & Römling, J. The impact of asymmetrical light input on cerebral hemispheric specialization and interhemispheric cooperation. Nat. Commun. 3:696 doi: 10.1038/ncomms1699 (2012).